Interleukin 2 modulates thymic-derived regulatory T cell epigenetic landscape Foxp3 + CD4 + regulatory T (T reg ) cells are essential for preventing fatal autoimmunity and safeguard immune homeostasis in vivo. While expression of the transcription factor Foxp3 and IL-2 signals are both required for the development and function of T reg cells, the commitment to the T reg cell lineage occurs during thymic selection upon T cell receptor (TCR) triggering, and precedes the expression of Foxp3. Whether signals beside TCR contribute to establish T reg cell epigenetic and functional identity is still unknown. Here, using a mouse model with reduced IL-2 signaling, we show that IL-2 regulates the positioning of the pioneer factor SATB1 in CD4 + thymocytes and controls genome wide chromatin accessibility of thymic-derived T reg cells. We also show that T reg cells receiving only low IL-2 signals can suppress endogenous but not WT autoreactive T cell responses in vitro and in vivo. Our findings have broad implications for potential therapeutic strategies to reprogram T reg cells in vivo. Naturally occurring, thymus-derived Foxp3 + T reg cells represent a distinct lineage of CD4 + T cells which major role is to maintain self-tolerance [1] , [2] , [3] , [4] . Foxp3, a forkhead/winged helix X-linked transcription factor (TF), is the major lineage-specifying TF for these cells and is indispensable for their differentiation, long-term maintenance, and suppressive functions [5] , [6] , [7] . Functional loss of FOXP3 is associated with the rapid onset of fatal T cell-mediated autoimmunity, also known as the IPEX syndrome in humans (immune dysregulation, polyendocrinopathy, enteropathy, X-linked [8] ) and the Scurfy phenotype in mice [5] , [6] , [7] . Foxp3 is induced in thymocytes undergoing positive selection following T cell receptor (TCR) triggering [9] , [10] and additional signals such as IL-2, which stabilizes Foxp3 and the associated thymic-derived T reg cell program of differentiation [11] , [12] , [13] . The transcriptional regulation of Foxp3 is complex involving the cooperation with multiple additional TFs to enable and maintain T reg cell functional attributes [10] , [12] , [14] , [15] , [16] . Foxp3 therefore acts as an essential TF, which sustained expression is regulated by three intronic conserved non-coding sequence (CNS) elements (CNS1-3) [17] . CNS3 for instance, acts as a pioneer element in inducing the expression of Foxp3 while CNS2 is bound by IL-2-activated STAT5, directly enabling the stabilization of Foxp3 expression in T reg cells [18] , [19] . The lack of IL-2, its high affinity receptor chain IL-2Rα/CD25 or its transducing chain IL-2Rβ/CD122 [20] , lead to the development of wasting autoimmunity as a result of the loss of stable Foxp3 expression [5] , [6] , [7] and subsequent Foxp3 + T reg cells in the periphery [21] , [22] , [23] . While the Foxp3 TF is required to maintain peripheral T reg cell identity and functions, it is not sufficient per se to confer the functional attributes of T reg cells [12] , [16] , [24] , also consistent with two-thirds of the T reg cell transcriptional signature that cannot be induced by ectopic expression of Foxp3 in T conv cells [14] , [25] . Studies using Foxp3 Gfp knock-in/out reporter mice in which GFP +/+ thymocytes lacked functional Foxp3, showed that Foxp3 acts to amplify and fix pre-established molecular features of T reg cells acquired during thymic selection but prior Foxp3 expression [14] . Foxp3 Gfp/Gfp thymocytes exhibit CpG hypomethylation patterns characteristic of mature peripheral T reg cells [24] . Foxp3 also overwhelmingly binds to pre-existing genome-wide enhancers in thymocytes committed to become T reg cells during positive selection [26] . Altogether these findings suggest that TCR-induces epigenetic modifications independently of Foxp3 but likely to involve other transcriptional regulators predefining T reg cell identity. Two recent reports provided mechanistic evidence for this concept [27] , [28] by showing (i) that the epigenetic modifier SATB1 is essential in activating T reg cell-specific super-enhancers associated with Foxp3 and other T reg -cell signature genes in thymic precursor T reg cells [27] and (ii) that the methylation enzyme MLL4, which regulates the level of monomethylated H3K4 and chromatin interactions at putative gene enhancers, sets the enhancer landscape for Foxp3 induction via chromatin looping [28] . These studies represent important conceptual advances in our understanding of the molecular genetics underlying T reg cell-lineage commitment. However, other signals subsequent or concomitant to TCR triggering that may contribute to setting up the functional identity of Foxp3 + T reg cells are largely unknown. IL-2 is proposed to be essential in this process [12] , [19] , [21] , [29] , but it is believed to be through the stabilization of the Foxp3 TF. Since TCR signaling leads to CD25 upregulation on thymocytes, it is conceivable that IL-2 contributes to establishing thymic T reg cell identity in vivo. Herein, we isolate and characterize a mouse model, the Il2ra mut/mut mouse that bears a point mutation in the IL-2 receptor high affinity chain CD25 resulting in a selective and quantifiable decrease in response to only high affinity IL-2 signals, to test the hypothesis that IL-2 signals modulate T reg cell epigenetic and transcriptional identity, and subsequent suppressive functions in vivo. Our results suggest that IL-2, possibly through the positioning of the genome organizer SATB1, modulates thymic-derived T reg cell epigenetic identity prior to Foxp3 expression. T reg cells that integrate low IL-2 signals ( Il2ra mut/mut ) only repress endogenous but not WT autoreactive T cells, illustrating further the importance of IL-2 signaling for optimal T reg cell functions. These observations are consistent with the idea that altering T reg cell epigenetic identity, in addition to IL-2 capture and signaling, leads to more rapid autoimmunity, and further raise the possibility that epigenetic reprogramming of T reg cells at the time of their selection in the thymus could improve T reg cell functions in autoimmune patients. Isolation of a novel IL-2 receptor alpha point mutant mouse During experiments in Ccr2 −/− mice [30] obtained from the Jackson Laboratory (JacksLab) in 2009, referred to as Ccr2 − / − 2009 , we observed that CD4 + Foxp3 + T reg cells in primary and secondary lymphoid organs and blood, displayed low to no cell-surface expression of the IL-2Rα/CD25 compared to T reg cells from wild type (WT) B6 counterparts (WT) (Supplementary Fig. 1a ). 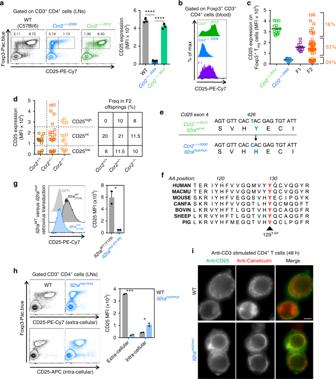Fig. 1 Isolation and characterization of theIl2ramut/mutmouse model.aLymph node cells isolated from WT,Ccr2−/−2009andCcr2−/−2012(all on the B6 background) mice were stained with mAbs against cell-surface CD3, CD4, CD25 (clone PC61), and intracellular Foxp3. A representative dot plot is shown. Bar graph summarizes CD25 expression levels (MFI) across all mice analyzed.bFACS histograms of cell-surface CD25 levels (MFI) gated on blood Foxp3+Tregcells (CD3+CD4+) fromCcr2−/−2009,Ccr2−/−2012, Ccr2+/−2009(F1) mice.cDistribution of CD25 cell-surface expression levels (MFI) in Tregcells from the blood of individual mice of indicated genotypes includingCcr2+/−2009×Ccr2+/−2009(F2) mice.dCcr2genotypes based on CD25 surface expression levels and experimental frequencies obtained in F2 offsprings.eDNA and corresponding amino-acid sequence alignments of the mutation found in exon 4 ofIl2ragene inCcr2−/−2009vsCcr2−/−2012mice after whole-exome sequencing.fAlignment of the CD25 amino-acid sequence surrounding tyrosine 129 across multiple species.gFACS histograms of cell-surface expression of CD25 in 293T cells retrovirally transduced with WT or mutagenized Y129HIl2racDNA. Bar graph shows CD25 expression (MFI) across two independent transduction experiments.hDot plots of cell-surface or intracellular expression levels (MFI) of CD25 in WT and mutant Tregcells. Bar graphs average data from one of 2–3 experiments with similar results with >2 mice per group.iFluorescent microscopy staining of CD25 on anti-CD3 stimulated purified CD4+T cells isolated from LNs. T cells were fixed and co-stained with anti-CD25 (green) and anti-calreticulin (red) prior to image acquisition. Scale bar is 5 μm.p-values are indicated when relevant with *p< 0.05; **p< 0.01; ***p< 0.001; NS not significant, using two-tailed unpaired Student’st-test. Error bars are mean ± SEM in all figures T reg cell frequency among CD4 + T cells was reduced in spleens and lymph nodes (LNs) while remaining comparable in blood and primary lymphoid organs (Supplementary Fig 1b, c ). Since Ccr2 − / − mice were neither reported to have different T reg cell frequencies nor distinct expression of CD25 compared to WT mice [31] , [32] , we re-acquired Ccr2 − / − mice from the JacksLab in 2012, referred to as Ccr2 − / − 2012 , and compared them to Ccr2 − / − 2009 mice (Fig. 1a ). As previously documented, and in contrast to Ccr2 − / − 2009 mice, T reg cell frequencies and CD25 expression were unaltered in Ccr2 − / − 2012 mice. We reasoned that the altered T reg cell phenotype could be accounted for by (i) a difference in the skin and/or gut microbiota between the two Ccr2 − / − lines, or (ii) a spontaneous mutation acquired in the Ccr2 − / − 2009 colony before 2009. Between 2009 and 2012, Ccr2 − / − 2009 mice were backcrossed twice to the WT B6 background and underwent 23 intercrosses (JacksLabs communication). Co-housing of Ccr2 − / − 2012 and Ccr2 − / − 2009 mice for 3 months neither rescued T reg cell frequencies nor expression of CD25 in Ccr2 − / − 2009 mice, likely ruling out a microbiota hypothesis (Supplementary Fig. 1d ). However, intercross of Ccr2 − / − 2009 and WT B6 mice revealed that T reg cells in the F1 offspring expressed twice as less cell-surface CD25 (MFI) compared to Ccr2 − / − 2012 T reg cells, but twice as more compared to Ccr2 − / − 2009 T reg cells, suggesting that the Ccr2 − / − 2009 trait is haploinsufficient (Fig. 1b, c ). Analysis of CD25 expression levels on T reg cells from 51 F2 offspring obtained from intercrossing F1 mice revealed a quasi-Mendelian distribution of the various possible phenotypes, consistent with the Ccr2 − / − 2009 trait being controlled by a single gene. Plotting CD25 expression as a function of CCR2 genotypes in the F2 progeny established that CCR2 and CD25 segregated independently of each other with the number of meiosis events close to 50% (Fig. 1d and Supplementary Fig. 1e ). This result suggests that the Ccr2 − / − 2009 trait depends on a single locus likely located on a distinct chromosome than the 9th that carries Ccr2 . Whole exome sequencing of Ccr2 − / − 2009 and Ccr2 − / − 2012 mouse DNA identified only 5 non-synonymous coding gene variants (Fig. 1e and Supplementary Fig. 1f ), with the most relevant coding variant replacing a single thymidine with a cytosine nucleotide on position 426 of exon 4 of the Il2ra gene in the Ccr2 − / − 2009 line. This mutation led to (i) the replacement of an evolutionarily highly conserved tyrosine (Y) with a histidine (H) on position 129 of the CD25 protein (Fig. 1f ), and (ii) the creation a new BssSI restriction site (Supplementary Fig. 1g ) which helped confirm the presence of this mutation in Ccr2 − / − 2009 but not Ccr2 − / − 2012 mice. Targeted mutagenesis of the Y129 of WT Il2ra to H129 and retroviral transduction of WT and H129 CD25 in 293T cells (Fig. 1g ) recapitulated the CD25 cell-surface expression phenotypes reported in Ccr2 − / − 2009 vs Ccr2 − / − 2012 mice, demonstrating that this point mutation accounted for the mouse phenotype. We next bred mice carrying only the homozygous Y129H mutation from the Ccr2 +/+ F2 progeny (Fig. 1c ), further referred to as Il2ra mut/mut mice. Fig. 1 Isolation and characterization of the Il2ra mut/mut mouse model. a Lymph node cells isolated from WT, Ccr2 − / − 2009 and Ccr2 − / − 2012 (all on the B6 background) mice were stained with mAbs against cell-surface CD3, CD4, CD25 (clone PC61), and intracellular Foxp3. A representative dot plot is shown. Bar graph summarizes CD25 expression levels (MFI) across all mice analyzed. b FACS histograms of cell-surface CD25 levels (MFI) gated on blood Foxp3 + T reg cells (CD3 + CD4 + ) from Ccr2 − / − 2009 , Ccr2 − / − 2012 , Ccr2 +/ − 2009 (F1) mice. c Distribution of CD25 cell-surface expression levels (MFI) in T reg cells from the blood of individual mice of indicated genotypes including Ccr2 +/ − 2009 × Ccr2 +/ − 2009 (F2) mice. d Ccr2 genotypes based on CD25 surface expression levels and experimental frequencies obtained in F2 offsprings. e DNA and corresponding amino-acid sequence alignments of the mutation found in exon 4 of Il2ra gene in Ccr2 − / − 2009 vs Ccr2 − / − 2012 mice after whole-exome sequencing. f Alignment of the CD25 amino-acid sequence surrounding tyrosine 129 across multiple species. g FACS histograms of cell-surface expression of CD25 in 293T cells retrovirally transduced with WT or mutagenized Y129H Il2ra cDNA. Bar graph shows CD25 expression (MFI) across two independent transduction experiments. h Dot plots of cell-surface or intracellular expression levels (MFI) of CD25 in WT and mutant T reg cells. Bar graphs average data from one of 2–3 experiments with similar results with >2 mice per group. i Fluorescent microscopy staining of CD25 on anti-CD3 stimulated purified CD4 + T cells isolated from LNs. T cells were fixed and co-stained with anti-CD25 (green) and anti-calreticulin (red) prior to image acquisition. Scale bar is 5 μm. p -values are indicated when relevant with * p < 0.05; ** p < 0.01; *** p < 0.001; NS not significant, using two-tailed unpaired Student’s t- test. Error bars are mean ± SEM in all figures Full size image Since the Y129H change impaired cell-surface expression of CD25 on T reg cells, we further hypothesized that CD25 may not be properly folded and/or lack stability. Based on the structure of human CD25, which has ~60% percent homology with mouse CD25, the Y129 likely makes stabilizing hydrogen bonds with a section of CD25 that is in direct contact with IL-2 (Supplementary Fig. 1h ). Consistent with this possibility, intracellular staining for CD25 revealed high levels of CD25 inside T reg cells from Il2ra mut/mut compared to WT mice, a finding also confirmed in retrovirally transduced 293T cells (Fig. 1h and Supplementary Fig. 1i ). CD25 subcellular localization in anti-CD3-stimulated CD4 + T cells from either Il2ra mut/mut or WT mice, suggested that mutant CD25 mostly co-localized with calreticulin, an endoplasmic reticulum (ER) resident protein. A strong staining of the nuclear envelope, a subdomain of the ER, was observed in Il2ra mut/mut but not WT CD4 + T cells, suggesting that the Y129H mutation prevented proper folding of CD25 and subsequent egress from the ER to the cell surface (Fig. 1i ). Thus, we isolated and characterized a mouse mutant line with a point mutation in an evolutionarily highly conserved tyrosine of the high affinity IL-2 receptor alpha chain CD25, likely preventing its optimal folding and subsequent cell-surface expression. Il2ra mut/mut T cells exhibit impaired responses to IL-2 We next assessed whether impaired cell-surface expression of CD25 on T cells translates into decreased IL-2 binding and signaling. Using labeled IL-2 incubated with anti-CD3 stimulated CD4 + T cells, we found higher IL-2 binding to WT compared to either Il2ra mut/mut or WT T cells incubated with an excess of non-biotinylated IL-2 (Fig. 2a and Supplementary Fig. 2a ). STAT5a phosphorylation, a very early signaling response that follows IL-2 binding to CD25, was also profoundly altered both in T reg cells from thymus and LNs and in conventional CD4 + T (T conv ) cells from Il2ra mut/mut mice (Fig. 2b and Supplementary Fig. 2a, b ). Consistent with these findings, Il2ra mut/mut CD8 + and CD4 + T conv cells proliferated substantially less compared to WT counterparts as quantified in vitro by CTV dilution of labeled T conv cells after anti-CD3 and varied amounts of IL-2 (Fig. 2c and Supplementary Fig. 2a, c ). To extend findings in vivo, we next monitored CD25 upregulation on K b /Ova 257-264 tetramer + (Tet + ) CD8 + T conv cells primed in WT or Il2ra mut/mut mice infected intravenously (i.v.) with Listeria monocytogenes expressing the model antigen Ovalbumin ( Lm-Ova ) (Fig. 2d ). Expression of CD25 by Ova-specific Tet + CD8 + T conv cells was lower in Il2ra mut/mut compared to WT mice [33] , in line with the in vitro data (Fig. 2d ). Then, we generated mixed bone-marrow chimeras from lethally irradiated recipient mice reconstituted with WT and Il2ra mut/mut donor bone-marrow cells (ratio 1:1) so that we could monitor and compare WT and Il2ra mut/mut antigen-specific CD8 + T conv cell responses in the same host (Fig. 2e and Supplementary Fig. 2d ). Reconstituted chimeras were further infected with Lm-Ova or the Herpes Simplex Virus 2 (HSV-2) intravaginally (i.vag. ), and both K b /Ova 257-264 and K b /gB 498-505 Tet + T conv cells were monitored at the peak of the primary response. In both models, Ova- and gB-specific Il2ra mut/mut CD8 + T conv cells expanded ~3-fold less than WT counterparts. Thus, the CD25 Y129H mutation profoundly alters CD25 expression and functional response to IL-2 in both T conv and T reg cells. Fig. 2 The Y129H mutation in CD25 impairs IL-2 binding, signaling and T cell proliferation. a Recombinant human IL-2 was biotinylated and incubated with anti-CD3 stimulated purified CD4 + T cells from Il2ra mut/mut or WT mice prior to staining with streptavidin PE. Unbiotinylated IL-2 was added to WT T cells as a control of binding specificity. Representative FACS histograms of IL-2 or no IL-2 bound to mutant or WT T cells are shown. The graph plots IL-2 binding signals (MFI) with increasing concentration of biotinylated IL-2. IL-2 Kd (50% binding capacity) for Il2ra mut/mut or WT T cells are shown. b Purified CD4 + T cells from LNs of Il2ra mut/mut or WT mice ( n = 3) were incubated in serum-free media (30’) and with IL-2 (20’) before proceeding to intracellular STAT5 phosphorylation staining. FACS histograms of STAT5 phosphorylation levels in Foxp3 + T reg (left) and anti-CD3 activated CD4 + T conv (right) cells are shown. Graphs plot phosphorylated STAT5 expression with increased IL-2 concentrations. c Purified LN CD4 + or CD8 + T cells from Il2ra mut/mut or WT mice were CFSE-labeled and incubated with anti-CD3 and IL-2. The proportion of CFSE low T cells was determined by FACS 4 days later. Graphs plot the % CFSE low T cells as IL-2 increases in 1 of 3 replicate experiments. FACS histograms show cell-surface CD25 expression in Il2ra mut/mut or WT T cells 4 days post IL-2 incubation. d Il2ra mut/mut or WT mice ( n = 2) were immunized i.v. with 10 4 WT Listeria monocytogenes (Lm) expressing Ovalbumin ( Lm -Ova) and spleen cells were stained at indicated days with Ova 257-264 /K d tetramers (Tet + ) and anti-CD25. Representative FACS histograms of CD25 expression on tet + CD8 + T cells is shown with a summary bar graph. e WT/ Il2ra mut/mut mixed bone-marrow (BM) chimeras (ratio 1:1) with discriminative CD45.1/2 congenic markers were immunized i.v. with WT Lm-Ova and 7.5 days later spleen cells stained with Ova 257-264 /K d tetramers. Representative FACS dot plots and summary bar graphs of Lm -specific Il2ra mut/mut or WT tet + CD8 + T cells are shown ( n = 15 mice). p -values are indicated with * p < 0.05; ** p < 0.01; *** p < 0.001; NS not significant, using two-tailed unpaired Student’s t -test. Error bars are mean ± SEM in all figures Full size image IL-2 modulates T reg cell epigenetic landscapes IL-2 signals are postulated to contribute to establishing the T reg cell program of differentiation before T reg cells express Foxp3 in the thymus [11] , [12] , [13] , [34] but only little evidence exist to support this hypothesis. To explore this possibility, we took advantage of the Il2ra mut/mut mouse model in which T reg cells receive reduced IL-2 signals, and asked whether their chromatin accessibility differs just after they have committed to the T reg cell lineage (thymus) and in the periphery in the secondary lymphoid organs (LNs). We isolated Foxp3 + T reg cells from thymus and LNs of Il2ra mut/mut and WT Foxp3 Rfp/Rfp reporter mice and conducted an analysis of the genome-wide open chromatin regions (OCRs) using an assay for transposase accessible chromatin with high-throughput sequencing (ATAC-seq [35] , Fig. 3 and Supplementary Fig. 3 ). While we found 36,200 and 32,369 OCRs (ATAC-seq peaks) in WT and Il2ra mut/mut thymic T reg cells respectively, LN T reg cells exhibited 25,167 and 24,639 OCRs (Fig. 3a ). Ninety-five percent of WT LN T reg cell OCRs identified overlapped with those reported in a prior study analyzing LN T reg cell OCRs [36] (Supplementary Fig. 3a ). As expected, this overlap was lower (75-80%) when we compared WT T reg cell’s OCRs to that reported in CD8 + T cells [37] . Within the thymic and LN T reg cell OCRs, we respectively identified 8031 and 8484 differentially accessible OCRs in WT (5931 in thymus and 4506 in LN) and Il2ra mut/mut (2100 in thymus and 3978 in LN) T reg cells (Fig. 3a ). This represents ~41% difference in the epigenetic landscape of WT vs Il2ra mut/mut LN T reg cells, which is comparable to what is reported between resting and activated T reg cell OCRs [36] (~36%, Supplementary Fig. 3b ). These differences are also similar to those measured between effector and memory or exhausted CD8 + T cells (34–41%) [37] , [38] , [39] but substantially greater than that reported in effector cells isolated from mice infected with acute vs chronic LCMV (~15%) [38] . Analysis of the relative localizations of differential OCRs in relation to the mouse ensemble annotated genes revealed a lower proportion of OCRs in the transcription start sites (TSS, ≤1 kb) compared to that of the overlapping peaks both for thymic and LN T reg cells (~9–14% vs 37–48%, Fig. 3b, c and Supplementary Fig. 3c and Data 1 ). The majority of unique peaks were found in introns and distal intergenic regions (>10 kb), suggesting that IL-2 signals regulate chromatin opening of elements distal to the TSS already at early stages of T reg cell commitment in the thymus. Upon assigning these peaks to the closest gene TSS, 651 (thymus) and 762 (LN) genes with differential OCRs were common to WT and Il2ra mut/mut T reg cells while the remaining were within non-overlapping genes (Fig. 3d and Supplementary Data 2 ). Approximately three times as many genes and OCRs were uniquely present in WT compared to Il2ra mut/mut thymic T reg cells (3401 vs 1107 genes) while LN T reg cells had comparable numbers of unique genes and OCRs (2356 vs 1992 genes)(Fig. 3a,d ). This result shows that the ratio of differential OCRs between WT and Il2ra mut/mut T reg cells from the thymus to the LNs is substantially modulated (from ~3:1 to 1:1), suggesting further functional commitment of T reg cells. Analysis of the biological-process (BP) gene-ontology (GO) pathways of genes containing unique peaks (<20 kb from TSS) in WT thymic and LN T reg cells highlighted a much greater diversity of BP (251 and 356 GO pathways vs only 86 and 14 GO pathways, respectively)(Fig. 3e and Supplementary Data 3 ). Since the differences in the number of genes with unique peaks between WT and Il2ra mut/mut T reg cells is much smaller compared to that of the GO pathways (Fig. 3d, e ), it further suggests that the OCRs in Il2ra mut/mut T reg cells are more random. While some processes related to T cell activation and tolerance are common to both types of T reg cells in the thymus, others targeting activation, migration and effector mechanisms are only maintained in WT LN T reg cells (Fig. 3f ). Conducting the GO pathway analysis on genes containing unique peaks without any limit from TSS revealed the exact same trend (Supplementary Fig. S3d,e and Data 3 ). Thus, IL-2 signals have a broad impact on genome-wide T reg cell epigenetic landscape, both for the opening and the closing of mostly TSS-distant regulatory regions. IL-2-mediated alterations occur already at early stages of T reg cell commitment to this lineage in the thymus and are sustained throughout LN T reg cells. Fig. 3 IL-2 makes substantial modifications in the epigenetic landscape of T reg cells: T reg cells (5 × 10 4 ) were sorted by flow cytometry from thymus or LNs of Il2ra mut/mut and WT Foxp3 Rfp/Rfp reporter mice, lysed and DNA from nucleus extracted for analysis of open chromatic regions by ATAC-seq. a Venn diagram of number of common and unique ATAC-seq peaks (OCRs) in Il2ra mut/mut vs WT T reg cells from thymus and LNs. b , c Distribution of common and unique ATAC-seq peaks across gene organization ( b ) and distance to the transcription start site (TSS, c ) in the whole genome. d , e Venn diagrams of number of genes ( d ) and GO pathways ( e ) exhibiting unique peaks in Il2ra mut/mut vs WT thymic and LN T reg cells on all ( d ) or within ( e ) 20 kb from TSS. f Network analysis of biological-process GO term enrichment among genes with unique peaks within 20 kb from TSS in Il2ra mut/mut or WT thymic and LN T reg cells. Genes were analyzed for over-represented GO terms using ReviGO. Node color is proportional to the FDR-adjusted p -value of the enrichment. Node size is proportional to gene set size Full size image IL-2-driven epigenetic changes mildly alter gene expression Since IL-2 induces extensive modifications in the chromatin of T reg cells (Fig. 3 ), we next assessed whether these alterations translated into a distinct program of expression between Il2ra mut/mut and WT LN T reg cells. The lack of IL-2 signaling in T reg cells was reported to only alter a relatively focused set of genes implicated in cell growth, metabolism, motility and adhesion, preventing their overall competitive fitness in vivo [21] , [29] , [40] . We purified total RNA from flow-sorted Foxp3 + (RFP + ) T reg or naive (CD62L hi CD44 lo ) T conv cells isolated from the LNs of WT or Il2ra mut/mut Foxp3 Rfp/Rfp reporter mice, and analyzed gene expression using microarrays (Fig. 4 ). While the expression profiles of naive T conv cells are almost identical between the two groups, that of Il2ra mut/mut and WT T reg cells exhibit significantly more differences (Fig. 4a and Supplementary Fig. 4a and Data 4 ). We note a set of 277 differentially expressed genes among which 128 and 149 are up- or downregulated respectively in Il2ra mut/mut compared to WT T reg cells (Fig. 4b and Supplementary Fig. 4b ). These genes are involved in cellular adhesion and cytoskeleton rearrangement, cell division and differentiation, cytokines and receptors, cellular activation and chemotaxis (Fig. 4c ), consistent with prior reports [21] , [29] , [40] . We checked some of the differentially upregulated genes for which Abs specific for encoded proteins are available, and found a direct correlation with protein expression levels for KLRG1, TIGIT, CCR4 while we did not for CCR5 or BTLA (Supplementary Fig. 4c ). Interestingly, increased expression of these markers is detected only in a small subset of CD4 + T reg cells, suggesting that lowering IL-2 signals promotes the onset of a subpopulation of T reg cells with a slightly distinct expression program, rather than altering the whole T reg cell population. Since only a few of the downregulated genes encode for proteins of known functions, we next focused primarily on sets of upregulated genes to run a comparison against known BP-GO databases (Fig. 4d and Supplementary Fig. 4d,e and Data 5 ). We found statistically over-represented gene sets implicated in cell adhesion, activation, proliferation/cell cycle, cellular differentiation as well as inflammatory processes, transcriptional regulators and chromatin organization/epigenetic gene regulation. While only a limited set of genes are differentially expressed in Foxp3 + T reg cells that receive lower IL-2 signals, the biological functions that are altered seem to directly target their ability to migrate, undergo homeostatic proliferation and express suppressive effector functions. We also noted differences in expression of genes implicated in various steps of chromatin modifications (Supplementary Fig. 4f ). Fig. 4 The expression of only a small set of genes in T reg cells is altered by low IL-2 signals: a 5 × 10 4 T reg and T conv cells were sorted by flow cytometry from LNs of three independent replicate Il2ra mut/mut or WT Foxp3 Rfp/Rfp reporter mice and total RNA extracted and reverse transcribed to cDNA. Affymetrix mouse expression arrays (Pico 1.0) were then conducted. Principal component analysis (PCA) of expressed genes using the top 10% of genes with the highest variance in analyzed groups with each symbol featuring one mouse. b Scatter plot of individual genes expressed in Il2ra mut/mut vs WT T reg cells. Significantly upregulated and downregulated genes, defined as genes with at least 1.5 fold change, p -value ≤ 0.01, are colored blue or black, respectively, and numbers are shown. c Heat map of selected genes grouped under various categories as indicated and for which expression is significantly different between Il2ra mut/mut and WT T reg cells. d Network analysis of biological-process gene-ontology (GO) term enrichment among significantly upregulated genes in Il2ra mut/mut vs control WT T reg cells. Upregulated genes were analyzed for over-represented GO terms using BiNGO in Cytoscape, and the resulting network was calculated and visualized using EnrichmentMap. Groups of similar GO terms were manually circled. Line thickness and color are proportional to the similarity coefficient between connected nodes. Node color is proportional to the FDR-adjusted p-value of the enrichment. Node size is proportional to gene set size. e Venn diagram comparing differentially expressed genes in Il2ra mut/mut vs WT T reg cells to genes with unique peaks called in Il2ra mut/mut and WT T reg cells found in ATAC-seq in Fig. 3 based on gene symbols. f ATAC-seq tracks for 3 sample genes with at least 1 unique peak localized in distinct regions of the gene (promotor, intronic, intergenic). g Three-way Venn diagram comparing differentially expressed genes in Il2ra mut/mut versus WT T reg cells to genes containing unique peaks close to TSS (<500 bp) in Il2ra mut/mut vs WT T reg cells found in ATAC-seq Full size image Most interestingly, although the number (4875) and relative proportion (~40%) of differential OCRs between Il2ra mut/mut and WT LN T reg cells is important (Fig. 3 ), those of differentially expressed genes (266) remain very small (below 1% of genes), suggesting that IL-2 signals play a more prominent role in shaping the epigenetic landscape and identity of T reg cells than their ability to express sets of genes (Fig. 4e and Supplementary Data 6 ). Among the differentially expressed genes, only 72 exhibited unique OCRs in either WT or Il2ra mut/mut LN T reg cells. These OCRs may contribute to the changes in gene expression via chromatin structure modifications while the remaining genes (194) are likely to be controlled at the level of gene transcription with no changes in chromatin structures. For instance, CD80 that is highly expressed in Il2ra mut/mut compared to WT LN T reg cells, exhibits greater OCRs heights in Il2ra mut/mut vs WT T reg cell promoter regions (Fig. 4f ). Differential OCRs are further noted in intergenic regions of KLRG1 or in intronic regions for TIGIT. Interestingly, neither the Foxp3 nor the Helios genes had differential OCRs between Il2ra mut/mut and WT T reg cells (Supplementary Fig. 4g and Data 7 ). Analysis of the potential binding motifs for TFs in the differential OCRs revealed that a different set of TFs such as FOXO and KLF family members, could possibly bind in WT but not Il2ra mut/mut T reg cells (Supplementary Fig. 4h ). Because chromatin structures in the vicinity of TSS regions play critical roles in the expression status of the gene, we tested if differentially expressed genes contain differential OCRs close to the TSS (Fig. 4g and Supplementary Data 6 ). Eleven differentially expressed genes contain differential OCRs close to their TSS (±500 bp) while the majority of the remaining genes did not, suggesting that these genes undergo epigenetic modifications mostly occurring on elements distal to the TSS such as gene enhancer regions. In summary, despite establishing major genome wide changes of the T reg cell epigenetic landscape, IL-2 signals on LN T reg cells at steady state only translate in modest modifications of their gene expression profiles. IL-2 regulates SATB1 positioning prior T reg cell commitment We next investigated how IL-2 signals mediate such large genome-wide changes in the T reg cell epigenome. Given its essential role in T reg cell-lineage specification and functions [5] , [6] , [7] , [14] , and its dependence on IL-2 [19] , [21] , one obvious candidate is the Foxp3 TF. If Foxp3 accounted for our observations, we predicted that Foxp3 binding regions would exhibit a very large overlap with the OCRs found in WT T reg cells but less with that of Il2ra mut/mut T reg cells (Supplementary Fig. 5a ). By aligning published chromatin immunoprecipitation sequencing (ChIP-seq) results of the Foxp3 TF defining the Foxp3 binding sites throughout the genome of LN T reg cells [26] with our ATAC-seq data, we found that Foxp3 DNA binding regions largely overlapped with OCRs common between Il2ra mut/mut and WT LN T reg cells, suggesting that IL-2-mediated alterations of the T reg cell epigenome are independent of Foxp3. Robust experimental evidence supports the idea that T reg cell epigenetic and functional identity is established in the thymus prior T reg cells express Foxp3 [13] , [24] , [25] , [26] . Notably, the pioneer factor SATB1 was reported to be essential for T reg cell-lineage specification before expression of Foxp3 in the thymus but not after [27] . Thus, we hypothesized that IL-2 acts through SATB1 before thymocytes commit to the T reg cell fate, at the single positive (SP) CD4 + thymocyte stage [11] , [13] , [24] . We know (Fig. 3 ) that mature Foxp3 + Il2ra mut/mut thymic T reg cells already exhibit differential OCRs compared to WT counterparts, suggesting epigenetic changes may have occurred before this stage. We conducted ChIP-seq experiments of SATB1 on SP CD4 + thymocytes isolated from Il2ra mut/mut or WT mice, postulating that SATB1 DNA positioning would differ if indeed this pioneer factor is involved in the regulation of IL-2-mediated T reg cell epigenetic changes (Fig. 5 ). The vast majority of SATB1-bound regions in WT and Il2ra mut/mut SP CD4 + thymocytes overlapped. While only 123 unique DNA regions are bound by SATB1 in WT thymocytes, SATB1 associate to more than 50% additional regions (2929) in Il2ra mut/mut thymocytes, showing that ectopic binding of this pioneer factor occurs when IL-2 signals are limiting (Fig. 5a ). Interestingly, the 123 unique SATB1-binding regions in WT thymocytes localize closer to promoter areas compared to that of Il2ra mut/mut counterparts which are far from TSS (>100 kb) in distal intergenic regions (Fig. 5b, c and Supplementary Fig. 5b ). Assigning the 123 SATB1-bound regions to the nearest gene TSS highlighted 96 genes among which 26 are common to Il2ra mut/mut T reg cells despite different SATB1-bound areas (Fig. 5d and Supplementary Data 7 ). Interestingly, 29 of the 96 genes with unique SATB1-binding sites are located within less than 2 kb from the TSS, and a majority encodes for DNA remodeling proteins, cell cycle, signal transduction and metabolism (Supplementary Fig. 5c ). These genes exhibit variable levels of expression across thymocyte development [41] , in particular between the SP CD4 + thymocyte and thymic T reg cell stages, consistent with a possible regulatory role of their expression by promoter-bound SATB1. SATB1 binds ~20 times more genes (2236) in Il2ra mut/mut compared to WT thymocytes, illustrating its ectopic binding when IL-2 signals are limiting (Fig. 5d ). BP-GO analysis on the common genes between the two conditions revealed that SATB1 targets common processes (~21) involved in DNA remodeling, transcriptional regulation and metabolism (Fig. 5e and Supplementary Fig. 5d and Data 8a,b ). However, when IL-2 signaling is impaired, SATB1-associated genes are implicated in 83 additional processes that include immune cell activation, adhesion and differentiation, and may reflect less focused binding. A search for known TF binding motifs within the regions bound by SATB1 highlighted GATA3, RUNX1 and ETS1 among the top ones, which are all associated with the regulation of Foxp3 expression [15] , [17] , [42] , [43] (Fig. 5g ). These motifs are AT-rich, which represent SATB1 preferential binding motifs [44] . While no enriched motifs are revealed in the 123 unique regions of WT SP CD4 + thymocytes, all of the prior ones are found in the remaining WT and Il2ra mut/mut SATB1-bound regions. The proportion of these TF-binding motifs is enriched in peaks common with WT thymocytes, suggesting a more focused binding of SATB1 when normal IL-2 signals are received. Thus, IL-2 signals have a significant impact on where the pioneer factor SATB1 binds to DNA in SP CD4 + thymocytes, which is likely to contribute to IL-2 modulation of the Foxp3 + T reg cell epigenetic landscape. Fig. 5 Ectopic DNA binding of SATB1 in SP CD4 + thymocytes receiving low IL-2 signals: 2 × 10 6 SP CD4 + thymocytes were sorted in 2 independent duplicate experiments by flow cytometry from the thymus of Il2ra mut/mut and WT mice, PFA fixed, lysed, and cross-linked DNA was used for chromatin immunoprecipitation sequencing (ChIP-seq) of the pioneer factor SATB1. a Venn diagram of the number of common and unique SATB1 DNA binding peaks in Il2ra mut/mut vs WT SP CD4 + thymocytes. b , c Distribution of common and unique SATB1 DNA binding peaks across gene organization ( b ) and distance to the transcription start site (TSS, c ) in the whole genome. d Venn diagram of the number of genes exhibiting unique SATB1 DNA binding peaks in Il2ra mut/mut vs WT SP CD4 + thymocytes. e Venn diagram of biological-process gene-ontology (BP-GO) from genes with unique SATB1 DNA binding peaks in WT vs Il2ra mut/mut SP CD4 + thymocytes. f Network analysis of BP-GO term enrichment among genes with unique SATB1 DNA binding peaks in WT SP CD4 + thymocytes. Genes with unique SATB1-binding peaks were analyzed for over-represented GO terms using BiNGO in Cytoskape, and the resulting network was calculated and visualized using EnrichmentMap in Cytoscape. Groups of similar GO terms were manually circled. Line thickness and color are proportional to the similarity coefficient between connected nodes. Node color is proportional to the FDR-adjusted p -value of the enrichment. Node size is proportional to gene set size. g Frequency of known TF binding site motifs enriched in common and unique SATB1 DNA binding peaks in WT and Il2ra mut/mut SP CD4 + thymocytes. Motif frequency (%) is shown in heat map Full size image Il2ra mut/mut mice lack autoimmunity despite altered chromatin Given the importance of IL-2 in T reg cell stability, immune homeostasis [21] , [22] , [23] , [40] and epigenetic programming (Figs. 3 , 5 ), we postulated that Il2ra mut/mut mice may develop symptoms consistent with autoimmunity over time. Monitoring of T cell phenotypes in the peripheral blood of Il2ra mut/mut and WT mice over ~1.5 years did not reveal any differences in cell-surface expression of classical activation markers (CD44, CD62L, KLRG1), in contrast to T cells from Foxp3 y/ − mice analyzed 1.5 months post birth (Fig. 6a and Supplementary Fig. 6a ). No T cell infiltrates were detected in the liver, pancreas or small intestine of Il2ra mut/mut mice, which all represent peripheral organs often associated with the onset of an autoimmune reaction (Fig. 6b ). We next investigated how mutant T reg cells may control autoreactive T conv cells and maintain immune homeostasis. We first conducted an extensive characterization of T reg cells from Il2ra mut/mut compared to WT mice (Fig. 6c and Supplementary Fig. 6b ). Il2ra mut/mut T reg cells express higher cell-surface levels of IL-7 and IL-15 survival receptors (CD127 and CD122) and lower levels of IL-15Rα, consistent with the idea that T reg cells receiving lower IL-2 signals may rely on the use of compensatory IL-7 and IL-15 cytokines [11] , [19] , [29] . These T reg cells also undergo increased cell proliferation (Ki67 + ) and upregulated T cell inhibitory receptors (CTLA4, GITR) and ICOS, which are reported to promote efficient T reg cell-mediated suppression [45] . We did not detect any difference in TCR Vβ usage (Supplementary Fig. 6c ), likely ruling out major biases in Il2ra mut/mut T reg cell repertoire. Since the common IL-2/IL-15 transducing beta chain CD122 was significantly upregulated on Il2ra mut/mut T reg cells compared to WT counterparts (spleen and thymus), we next crossed Il2ra mut/mut mice to Il15 − / − mice, postulating that IL-15 signals are essential for mutant T reg cells to maintain immune homeostasis in these mice (Fig. 6d ) and compensate for impaired IL-2 signals though Il2ra mut/mut mice have higher levels of circulating IL-2 (Supplementary Fig. 6d ). The proportion of activated CD4 + (CD62L lo CD44 hi ) and CD8 + (CD62 lo KLRG1 + ) T conv cells in Il2ra mut/mut Il15 − / − and Il15 − / − mice was equivalent (Fig. 6d ) and similar to that of WT mice (Fig. 6a ), but significantly lower than in Foxp3 y/ − mice. In addition, we did not find any evidence of T cell infiltrates in the liver or the spleen of these mice (Supplementary Fig. 6e ). However, the proportion of Foxp3 + T reg cells in Il2ra mut/mut Il15 − / − mice was reduced compared to WT, Il2ra mut/mut or Il15 − / − mice (Fig. 6e ). Recently, two distinct subsets of T reg cells discriminated on CD44, CD62L and CCR7 expression were proposed to require either IL-2 (CD44 lo CD62 hi ) or ICOS (CD44 hi CD62 lo ) signaling for their maintenance [46] . Since we noted high cell-surface expression of ICOS on Il2ra mut/mut T reg cells (Fig. 6c ), we reasoned that impaired IL-2 signals might favor the onset of a CD44 hi CD62 lo T reg cell subset that requires ICOS signaling. Unexpectedly, we only observed lower proportions of the CD44 hi CD62 lo T reg cell subset in Il2ra mut/mut and Il2ra mut/mut Il15 − / − compared to WT mice, and this proportion was even further decreased by blocking ICOS for 2 weeks (Fig. 6f ). The overall proportion of Foxp3 + T reg cells among CD4 + T cells in the blood of ICOS-neutralized Il2ra mut/mut Il15 − / − mice was also reduced by ~50%, although mice did not develop autoimmunity (Fig. 6e and Supplementary Fig. 6f ), suggesting that none of the proposed mechanisms accounts for the absence of autoimmune disease in Il2ra mut/mut mice. Fig. 6 Il2ra mut/mut mice do not develop any signs of autoimmunity: a T cells collected from blood of Il2ra mut/mut and WT mice were stained for cell-surface CD3, CD8, CD4 and CD62L, CD44, KLRG1 activation markers at indicated times over an 18 months period. Blood from control Foxp3 y/ − was analyzed at ~1.5 months post birth. Each symbol represents an individual mouse. b At month 18, liver, pancreas, and small intestine were harvested, fixed/cut, and stained with H/E. c Spleen cells from 8 to 10-weeks-old Il2ra mut/mut and WT mice were stained for cell-surface CD3, CD4, intracellular Foxp3 and indicated markers. Overlay of representative FACS histograms after gating on CD3 + CD4 + Foxp3 + T cells are shown and bar graphs average relative expression levels (MFI, n = 4–5). d Blood from Il2ra mut/mut Il15 − / − , Il15 − / − (6 months old) or Foxp3 y/ − mice was stained as in a and representative FACS dot plots with bar graphs summarizing average across mice ( n = 6–7) are shown. e Proportion of peripheral blood Foxp3 + T reg cells among CD3 + CD4 + T cells in indicated mice treated (or not) with anti-ICOSL for 2 weeks. f Blood leukocytes from indicated mice groups were stained for expression of CD3, CD4, intracellular Foxp3, CD62L, CD44. Representative dot plots and summary bar graphs of average CD44/CD62L expression levels across all groups of mice are shown ( n = 3–4). p -values are indicated when relevant with * p < 0.05; ** p < 0.01; *** p < 0.001; NS not significant, using two-tailed unpaired Student’s t- test Full size image Il2ra mut/mut T reg cells cannot repress WT autoimmune T cells Lack of IL-2 or its receptor chains leads to fatal autoimmunity because T reg cells are unstable and fail to suppress autoreactive T conv cells [11] , [12] , [13] . Yet, mice in which IL-2 signaling is genetically altered by targeted mutation in the IL-2Rβ/CD122 transducing chain do not become autoimmune [29] . Thus, we reasoned that similar to IL-2Rβ mutant T reg cells, Il2ra mut/mut T reg cells may repress Il2ra mut/mut but not WT autoreactive T conv cells. As a first step to assess this idea, we conducted a standard in vitro suppression assay using increasing numbers of Il2ra mut/mut or control WT T reg cells incubated with CFSE-labeled anti-CD3 activated T conv cells (Supplementary Fig. 7a ). Il2ra mut/mut T reg cells inhibit T conv cell proliferation ~two fold less than WT T reg cells across all ratios, possibly accounting for the lack of autoimmunity in Il2ra mut/mut mice. Since T reg cells grown in vitro with anti-CD3/CD28 stimulation and under limited IL-2 availability lose Foxp3 expression and convert to effector T cells [18] , we next assessed whether Il2ra mut/mut T reg cells also lacked stability after TCR triggering in vitro (Supplementary Fig. 7b ). While ~60% of WT T reg cells lost Foxp3 expression, ~85% of Il2ra mut/mut converted to Foxp3 neg T cells, consistent with impaired lineage stability when IL-2 signals are limiting. Thus, even if they can prevent autoimmunity in Il2ra mut/mut mice, Il2ra mut/mut T reg cells may not be able to suppress WT autoreactive T conv cells to the extent to which WT T reg cells can. To further evaluate their suppressive capacity in vivo, we used two distinct but complementary models of acute autoimmunity development, and a model of reconstitution at homeostasis. We first conducted rescue experiments of Foxp3 y/ − mice [5] which develop fatal autoimmunity within ~3–4 weeks post birth, by transferring T reg cells sorted from the secondary lymphoid organs (SLOs) of WT or Il2ra mut/mut Foxp3 Rfp/Rfp reporter mice to recipient neonates (day 1–3) (Fig. 7a ). As expected, Foxp3 y/ − mice receiving WT T reg cells survived, while those transferred with Il2ra mut/mut T reg cells did not control the development of wasting disease and ultimately succumbed, as did untransferred counterparts. Second, we adoptively transferred CD4 + CD25 neg T conv cells to Rag1 − / − mice, which also results in a rapid wasting disease unless functional T reg cells are co-transferred (Fig. 7b ). As predicted from the first model, Il2ra mut/mut T reg cells fail to suppress autoreactive T conv cell-mediated autoimmunity with a rapid loss of weight and massive infiltrates of T cells in multiple organs (lung, liver, small intestine) in contrast to control groups transferred with WT T reg cells or only CD4 + T conv cells (Fig. 7c and Supplementary Fig. 7c ). Consequently, the absolute numbers of CD4 + T conv cells were two (lung) to five (spleen) fold increased in autoimmune mice with a higher proportion secreting IL-2 (factor of 2), IL-17A, and IFNγ (Fig. 7d ). Fate mapping of Il2ra mut/mut or WT T reg cells transferred to Rag1 − / − (Fig. 7e ) or Foxp3 y/ − (Supplementary Fig. 7d ) mice further showed that Foxp3 + Il2ra mut/mut T reg cells become ex-T reg cells and are lost compared to WT counterparts, both in proportion and absolute numbers. Thus, a threshold of IL-2 signals to T reg cells is needed to program their functional attributes, for their maintenance, and to prevent wasting autoimmunity. Consistent with this conclusion and the lack of competitive fitness [21] of Il2ra mut/mut T reg cells, a significantly lower proportion of Il2ra mut/mut compared to WT T reg cells was measured in WT B6 chimeric mice reconstituted with an equal ratio of Il2ra mut/mut and WT bone-marrow donor cells while the proportion of CD4 + T conv cells was maintained (Fig. 7f ). Fig. 7 T reg cells receiving limited IL-2 signals cannot suppress autoreactive WT T conv cells: a Foxp3 y/ − Cd45.1 +/+ neonate mice were transferred i.p. with 10 6 Il2ra mut/mut or WT flow-purified Foxp3 Rfp/Rfp CD3 + CD4 + T reg cells and survival was monitored over 120 days. Graphs average results over multiple mice in each group and 7-16 replicate experiments. b , c Rag1 − / − mice received 5 × 10 5 flow-purified Foxp3 Rfp/Rfp CD3 + CD4 + T reg cells together with 1.5 × 10 6 WT CD3 + CD4 + CD25 neg T conv cells i.v. Weight loss was monitored up to 61 days post transfer and immune cell infiltrates on H/E stained sections is shown at day 61 ( n = 4). d Numbers of transferred Foxp3 Rfp/Rfp CD3 + CD4 + T reg cells in the spleen and lung of Rag1 − / − mice (left bar graphs) and proportion of cytokine-secreting CD3 + CD4 + T conv cells 4 h post PMA/ionomycin stimulation. e Foxp3 expression in Foxp3 Rfp/Rfp CD3 + CD4 + T reg cells 45 and 75 days post transfer, proportion and absolute numbers of ex-T reg cells in LNs and spleens. f , g Schematic of mixed bone-marrow chimera generation in lethally irradiated WT B6 recipient mice with discriminative congenic markers. f , g Representative FACS dot plots of Foxp3 and CD4 expression in blood T cells of f WT /Il2ra mut/mut and g Foxp3 y/ − /WT and Foxp3 y/ − /Il2ra mut/mut chimeras 10 and 6 weeks post reconstitution, respectively. Graph in f shows the ratio of WT vs Il2ra mut/mut T conv and T reg cells for each individual chimera. Data are across several chimeras (5–9 mice/group) in 3–4 replicate experiments. h , i Spleen, LN pictures, and H/E stained sections of lung, liver, pancreas, and small intestine from Foxp3 y/ − /WT and Foxp3 y/ − /Il2ra mut/mut chimeras. j Cells from indicated organs from the two groups of chimeras were stained for cell-surface expression of CD3, CD4, CD8, CD62L, KLRG1, and CD44. Bar graphs show the proportion of activated CD4 + (CD44 + CD62L lo ) or CD8 + (KLRG1 + CD62L lo ) T cells ( n = 5–9). k Proportion of activated CD3 + CD4 + or CD8 + T conv cells from Il2ra mut/mut or WT BM in Foxp3 y/ − /Il2ra mut/mut chimeras. Bar graphs summarize average proportion across mice ( n = 5–9). p-values are indicated when relevant with * p < 0.05; ** p < 0.01; *** p < 0.001; NS not significant, using two-tailed unpaired Student’s t -test. Symbols on bar graphs feature individual mice Full size image As a last step to assess Il2ra mut/mut T reg cells functional attributes, we created another chimeric mouse model at homeostasis in which T reg cells lacked full IL-2 responsiveness while T conv cells responded normally. We reconstituted lethally irradiated WT mice with bone marrow cells from Foxp3 y/ − and Il2ra mut/mut or control WT mice (Fig. 7g ). In such Foxp3 y/ − / Il2ra mut/mut chimeras, only T reg cells lacked CD25 expression and mice exhibited enlarged spleens and LNs compared to the Foxp3 y/ − /WT control chimeras (Fig. 7h ). Moreover, massive infiltrates of T cells were noted in lung, liver, pancreas and small intestine of Foxp3 y/ − / Il2ra mut/mut mice, with gross architectural tissue alterations compared to the control group (Fig. 7i ). In line with these findings, both CD4 + and CD8 + T cells in Foxp3 y/ − / Il2ra mut/mut but not Foxp3 y/ − /WT chimeras underwent robust activation (CD62L low , KLRG1 + , CD44 hi , CD69 hi ) across multiple tissues (Fig. 7j and Supplementary Fig. 7e, f ). Only WT but not Il2ra mut/mut T conv cells in Foxp3 y/ − / Il2ra mut/mut chimeras were activated (Fig. 7k and Supplementary Fig. 7g ), suggesting that equal responsiveness to IL-2 by T conv cells and T reg cells represent a major parameter safeguarding immune homeostasis. In summary, T reg cells that can only integrate lower IL-2 signals than their T conv cell counterpart, acquire a suboptimal epigenetic program, are less stable (Foxp3) and are impaired in their ability to deprive autoreactive T conv cells of IL-2. While the Foxp3 TF is required to maintain peripheral T reg cell identity and functions, it is not sufficient to secure their stable epigenetic identity and program their functional features [12] , [16] , [24] . But how exactly are T reg cell chromatin accessibility characteristics determined before Foxp3 is expressed is still hotly debated. TCR signaling represents the major cue driving thymic selection, and this plays a determining role in thymocytes commitment to the T reg cell lineage [47] , however this is likely not sufficient [12] , [14] , [25] . Signals such as IL-2 and TGFβ cytokines, are suggested to contribute to the epigenetic modeling of T reg cells [2] , [3] , yet current evidence for IL-2 mostly pointed to its role as a major stabilizer of Foxp3 expression. Here, our data support a role for IL-2 in defining the epigenetic identity of Foxp3 + T reg cells, which appears largely independent of Foxp3. In fact, genome-wide chromatin accessibility changes when IL-2 signals are impaired are much wider than the regions where Foxp3 binds. Our whole genome analysis of OCRs in Il2ra mut/mut vs WT T reg cells from the LNs reveals that the epigenetic landscapes are widely distinct (~41%). Consistent with this result, constitutive STAT5 expression, which forces IL-2 signaling, is shown to divert thymocyte selection to the T reg cell lineage [11] . Using data from a prior report on T reg cell epigenetic signature under various conditions of activation [36] , we analyzed that ~36% of OCRs differed in activated vs resting Foxp3 + T reg cells, a proportion comparable to the extent of IL-2-mediated remodeling observed in WT vs IL2ra mut/mut LN T reg cells. These differences are equivalent to what is documented between effector and memory or exhausted CD8 + T cells [38] , which are undergoing extensive chromatin remodeling upon differentiation [37] , [38] , [39] , overall supporting the conclusion that IL-2 signals significantly shape the epigenetic landscape of T reg cells in vivo. Because IL-2 signals mediate genome-wide chromatin remodeling beyond Foxp3, and already on mature Foxp3 + T reg cells in the thymus, we postulated that this may occur in the thymus at the SP CD4 + thymocyte stage preceding Foxp3 expression in committed T reg cells. The genome organizer SATB1, which is highly expressed during most stages of T cell thymic selection, was recently involved in setting-up thymic-derived T reg cell functional features and ability to prevent autoimmunity before Foxp3 is turned on [27] . We further reveal that SATB1 positioning in the genome of SP CD4 + thymocytes impaired in IL-2 signaling, is much broader than in WT thymocytes, likely reflecting ectopic binding of this pioneer factor when IL-2 signals are limiting. Our finding that more than 20 times as many GO pathways are associated with the genes exhibiting unique OCRs in WT LN T reg cells compared to IL2ra mut/mut counterparts supports the idea that such ectopic binding of SATB1 lead to unfocused T reg cell chromatin modeling. In WT thymocytes, SATB1 is more selectively bound to the TSS of genes encoding for TFs and nucleic acid binding proteins, which may in turn control the correct T reg cell epigenetic landscape. Several TFs such as STAT5 and PI3/MAP kinase-dependent TFs, are activated downstream of IL-2 signaling. From our analysis of the SATB1 DNA binding regions and TFs known to bind to these motifs, we noted GATA3, RUNX1 and ELF1 that are all reported to be present prior to Foxp3 expression to enable its future recruitment and optimal function [15] , [17] , [26] , [43] . SATB1 is also described among the “quintet” TFs—together with Foxp3—that are essential for in vitro re-programing of T conv cells to T reg cells [16] . While still speculative, it is possible that IL-2 signals, in addition to TCR triggering, are essential to promote the expression/activation of the previous TFs and of SATB1 and/or other pioneer factors, to set-up the appropriate epigenetic landscape on which Foxp3 and these partner TFs act to achieve the final T reg cell identity. Binding to the Foxp3 CNS3 and CNS2 elements for instance is essential to initiate and then stabilize expression of Foxp3 [17] , [18] , [26] , [48] . The NF-kB subunit c-Rel binds CNS3, and STAT5 and GATA3 [49] stabilize CNS2. While we did not find evidence for SATB1-binding on c-Rel or STAT5 motifs, SATB1 may associate with GATA3 to help focus its binding to DNA area relevant to the acquisition of the T reg cell signature prior Foxp3 is expressed. Such mechanism would prevent ectopic binding of SATB1 throughout the genome when IL-2 signals are limiting. The consequence of lower IL-2 signaling in thymic-derived peripheral T reg cells is a different epigenetic landscape, which we suggest is being set in the thymus through SATB1 together with other IL-2-dependent TFs. In the periphery, however, SATB1 is not required to sustain functional thymic-derived T reg cells [27] . Some TF binding motifs found in SATB1-binding regions like RUNX1, which is likely to interact with SATB1 in SP CD4 + thymocytes, are also among the motifs found in the differential OCRs of WT compared to Il2ra mut/mut T reg cells in the periphery. RUNX1 binds to the IL-2 promoter and promotes its transcription, but is repressed by Foxp3 through physical interactions [42] , preventing the expression of an effector T cell program by T reg cells. Other TF binding motifs only found in WT peripheral T reg cells, such as FOXO1 and FOXO3, also bind to the Foxp3 promoter and conserved intronic enhancer regions, allowing for Foxp3 expression and T reg cell-lineage specification [50] . IL-2-mediated induction of all these TFs at the pre-T reg cell stage, via SATB1 or not, may help maintain the T reg cell program in the periphery. Along these lines, we noted multiple differentially expressed TF-encoding genes ( Prdm1, Gata3, Dzip1, Irf4 ), chromatin remodeling- and histone-encoding genes between WT and Il2ra mut/mut LN T reg cells. Given that our data support a model in which IL-2 alters T reg cell epigenetic identity early during thymic selection when thymocytes commit to this lineage, it is unlikely that this mechanism will be at work for induced T reg cells in peripheral tissues [51] . Our analysis in WT vs Il2ra mut/mut T reg cells failed to reveal any differences in OCRs of genes encoding Foxp3 or HELIOS that were reported to exhibit differential methylation profiles in induced/peripheral T reg cells [52] . We report a role for IL-2 on Foxp3 + T reg cells that is largely independent of Foxp3-mediated stabilization of T reg cells and of their ability to capture IL-2 from activated T conv cells. The Y129H mutation in CD25 prevents optimal folding and/or egress of CD25 to the surface of T cells, translating into decreased binding of IL-2 and subsequent signaling and proliferative response. Two closely comparable models were previously reported: in the first, mutations inside several of key signal transducing cytoplasmic tyrosines of the IL-2Rβ chain disrupted both IL-2 or IL-15 signaling [29] . The second model overexpressed a constitutively active form of the b subunit of the STAT5 TF [51] on either IL-2Rβ ( Cd122 − / − ) [19] or IL-2Rγ ( γc − / − ) knockout backgrounds [11] . None of these models could differentiate between IL-2 and IL-15, or other γ-chain-dependent cytokine signaling, confounding interpretation on the roles of high affinity IL-2 signaling. Nevertheless, a rather intriguing finding in both of these settings, as in our model, is that receptor deficient mice did not develop autoimmunity, prompting the idea that T reg cells were set to a low IL-2 receptor signaling threshold sufficient for Foxp3 induction and maintenance. Our current results, however, favor a different interpretation in which, when comparable IL-2 signals are received by T reg and T conv cells, the development of autoimmunity can be prevented. Yet, if T reg cells cannot receive as much IL-2 signals as T conv cells, mice will develop fatal wasting disease. A third model recently developed by Rudensky and colleagues, enabled to discriminate the contribution of IL-2 capture and T reg cell stability in preventing fatal autoimmunity [40] . As T reg cells cannot secrete IL-2 [6] but constitutively express the high affinity IL-2Rα/CD25 chain, a large conundrum in the field is their reliance on cell-extrinsic IL-2 from activated -potentially autoreactive- T conv cells, thus preventing excessive T conv cell proliferation and activation by physically capturing the IL-2 they secrete. This study brought strong evidence that IL-2 capture does represent a key mechanism of suppression used by T reg cells. While the Il2ra mut/mut mouse does not allow to assess the role of IL-2 capture by T reg cells in maintaining immune homeostasis, the progression of disease and survival in Foxp3 y/ − mice rescued with Il2ra mut/mut T reg cells, the Rag − / − transfer experiments and the Foxp3 y/ − / Il2ra mut/mut chimeras, are close to that observed in Foxp3 y/ − mice. Length of survival is, however, distinct to that of the Rudensky model, in which mouse survival is approximately twice increased. In this latter model too, CD8 + but not CD4 + T cells, exhibit robust activation whereas in our Foxp3 y/ − / Il2ra mut/mut chimeras, both subsets of T conv cells are highly activated. Altogether, these observations support the idea that altering T reg cell epigenetic identity, IL-2 capture and signaling leads to more rapid autoimmunity. IL-2 therapy has been used for over two decades in patients, initially with the goal to boost anti-tumoral and HIV-specific immunity [52] , [53] . High doses of IL-2 were mostly used with important side effects and mitigated efficiencies. Yet the use of lower doses of IL-2, with the underlying rationale that T reg cells would be more efficiently targeted than effector T cells, showed a preferential expansion of T reg cells both in preclinical models and in type 1 diabetes patients, which was associated with better prognostic markers [54] , [55] . While the mechanism underlying these promising outcomes in patients may be accounted for by T reg cell expansion, our results further raise the possibility that qualitative changes at the levels of chromatin accessibility and epigenetic reprogramming of T reg cells during thymic selection, may contribute to ameliorate T reg cell functions in autoimmune patients. Ethics statement This study was carried out in strict accordance with the recommendations by the animal use committees at the Albert Einstein College of Medicine. All efforts were made to minimize suffering and provide humane treatment to the animals included in the study. Mice All mice were bred in our SPF animal facility at the Albert Einstein College of Medicine. We used wild-type (WT) C57BL/6J (B6) 6-8 weeks old mice, congenic CD45.1 +/+ (#2014), Ccr2 − / − 2009 (#4999) , Ccr2 − / − 2012 (#4999) , Foxp3 +/ − (#19933) , Foxp3 Rfp/Rfp (#8374) , Rag1 − / − (#2216) from the Jackson labs all on the B6 genetic background. Ccr2 +/+2009 Il2ra mut/mut (called Il2ra mut/mut ) were generated by intercrossing to the B6. Il15 − / − (#4269) mice were purchased from Taconic. Microbial pathogens and mice infections We used wild type Listeria monocytogenes expressing the Ovalbumin (Ova) model antigen ( Lm -Ova) on the 10403s genetic background [56] . For infections, bacteria were grown to a logarithmic phase in broth heart infusion medium, diluted in PBS to infecting concentration (10 4 ) and injected i.v. For Herpes Simplex Virus 2 (HSV-2) infection , female mice treated with 2 mg medroxyprogesterone acetate subcutaneously (s.c.) were immunized or not 5 days later intravaginally with 2 × 10 5 plaque forming units (PFU) of 186ΔKpn HSV-2 (TK − HSV-2) and organs (spleen and draining LNs) were harvested 7 days later. Cell suspensions for flow cytometry and adoptive transfers Spleens, lymph nodes (inguinal and cervical), or thymuses were dissociated on nylon mesh while lungs, liver, and pancreas were cut. All organs were incubated in HBSS medium with 4000 U/mL collagenase I and 0.1 mg/mL DNase I, and red blood cells (RBC) lysed with NH 4 Cl buffer (0.83% vol/vol). Blood was harvested into heparin tubes and RBC lysed as before. Bone marrow cells were obtained from flushing femur with complete RPMI with 10% FCS. Cell-staining for FACS analysis Cell suspensions were incubated with 2.4G2 Fc Block and stained with fluorescently tagged antibodies (Abs) purchased from eBioscience, BD Biosciences, Tonbo Bioscience, or BioLegend (Supplementary Table 1 ) in PBS 1% FCS, 2 mM EDTA, 0.02% sodium azide. Biotinylated monomers (1 mg/mL) obtained from the NIH tetramer Core Facility, were conjugated with PE-labeled Streptavidin (1 mg/mL) as follow: 6.4 μL of PE-Streptavidin were added to 10 μL of monomers every 15 min four times on ice. Newly generated tetramers (1/400-1/500 dilution) were then used to stain spleen/LN cells for 1 h at 4 °C. For transcription factor (TF) intracellular staining (Foxp3, Blimp-1), cells were fixed in eBioscience Fixation/Permeabilization buffer prior to TF Ab staining in eBioscience Permeabilization buffer for 30 min. For intracellular cytokine staining (ICS), cells were incubated 4 h at 37 °C/5%CO 2 in RPMI1640 10%FCS, Golgi Plug/Golgi Stop (BD), fixed in IC fixation buffer (eBioscience), and permeabilized prior to 30 min staining with Abs against indicated intracellular markers. For intracellular phosphorylated STAT5 staining, cells were starved in RPMI w/o FCS for 30 min before stimulation with variable concentration of recombinant human IL-2 (Gemini) for 20 min. 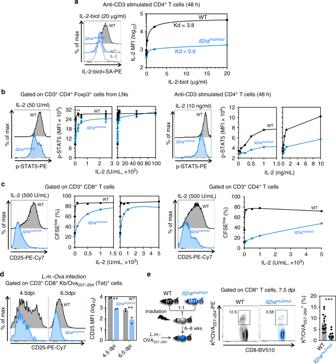Fig. 2 The Y129H mutation in CD25 impairs IL-2 binding, signaling and T cell proliferation.aRecombinant human IL-2 was biotinylated and incubated with anti-CD3 stimulated purified CD4+T cells fromIl2ramut/mutor WT mice prior to staining with streptavidin PE. Unbiotinylated IL-2 was added to WT T cells as a control of binding specificity. Representative FACS histograms of IL-2 or no IL-2 bound to mutant or WT T cells are shown. The graph plots IL-2 binding signals (MFI) with increasing concentration of biotinylated IL-2. IL-2 Kd (50% binding capacity) forIl2ramut/mutor WT T cells are shown.bPurified CD4+T cells from LNs ofIl2ramut/mutor WT mice (n= 3) were incubated in serum-free media (30’) and with IL-2 (20’) before proceeding to intracellular STAT5 phosphorylation staining. FACS histograms of STAT5 phosphorylation levels in Foxp3+Treg(left) and anti-CD3 activated CD4+Tconv(right) cells are shown. Graphs plot phosphorylated STAT5 expression with increased IL-2 concentrations.cPurified LN CD4+or CD8+T cells fromIl2ramut/mutor WT mice were CFSE-labeled and incubated with anti-CD3 and IL-2. The proportion of CFSElowT cells was determined by FACS 4 days later. Graphs plot the % CFSElowT cells as IL-2 increases in 1 of 3 replicate experiments. FACS histograms show cell-surface CD25 expression inIl2ramut/mutor WT T cells 4 days post IL-2 incubation.dIl2ramut/mutor WT mice (n= 2) were immunized i.v. with 104WTListeria monocytogenes (Lm)expressing Ovalbumin (Lm-Ova) and spleen cells were stained at indicated days with Ova257-264/Kdtetramers (Tet+) and anti-CD25. Representative FACS histograms of CD25 expression on tet+CD8+T cells is shown with a summary bar graph.eWT/Il2ramut/mutmixed bone-marrow (BM) chimeras (ratio 1:1) with discriminative CD45.1/2 congenic markers were immunized i.v. with WTLm-Ovaand 7.5 days later spleen cells stained with Ova257-264/Kdtetramers. Representative FACS dot plots and summary bar graphs ofLm-specificIl2ramut/mutor WT tet+CD8+T cells are shown (n= 15 mice).p-values are indicated with *p< 0.05; **p< 0.01; ***p< 0.001; NS not significant, using two-tailed unpaired Student’st-test. Error bars are mean ± SEM in all figures Cells were then fixed and permeabilized with 4% PFA followed by 90% methanol, and stained with anti-pY-STAT5 antibody (BD Biosciences). Data acquisition was done using a BD LSR II or a FACS Aria III flow cytometer. All flow cytometry data were analyzed using FlowJo v9 software (TreeStar). Cell sorting of Foxp3 + and Foxp3 − cells was performed based on RFP expression in Foxp3 Rfp/Rfp reporter mice using a BD FACS Aria III cell sorter. The FACS gating strategies for the experiments shown and T cell sorting are provided in Supplementary Fig. 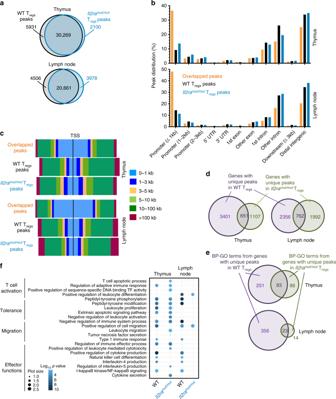Fig. 3 IL-2 makes substantial modifications in the epigenetic landscape of Tregcells: Tregcells (5 × 104) were sorted by flow cytometry from thymus or LNs ofIl2ramut/mutand WTFoxp3Rfp/Rfpreporter mice, lysed and DNA from nucleus extracted for analysis of open chromatic regions by ATAC-seq.aVenn diagram of number of common and unique ATAC-seq peaks (OCRs) inIl2ramut/mutvs WT Tregcells from thymus and LNs.b,cDistribution of common and unique ATAC-seq peaks across gene organization (b) and distance to the transcription start site (TSS,c) in the whole genome.d,eVenn diagrams of number of genes (d) and GO pathways (e) exhibiting unique peaks inIl2ramut/mutvs WT thymic and LN Tregcells on all (d) or within (e) 20 kb from TSS.fNetwork analysis of biological-process GO term enrichment among genes with unique peaks within 20 kb from TSS inIl2ramut/mutor WT thymic and LN Tregcells. Genes were analyzed for over-represented GO terms using ReviGO. Node color is proportional to the FDR-adjustedp-value of the enrichment. Node size is proportional to gene set size 8 . Transfection of wild-type and Y129H Il2ra in 293T cells The Il2ra cDNA was amplified by PCR and cloned into pMSCV-IRES-GFP (pMIG, kind gift from Guy Sauvageau) to generate pMIG- Il2ra . PCR was performed on pMIG- Il2ra to introduce a point mutation on nucleotide 426 (thymidine to a cytosine), which results in a tyrosine-histidine conversion at amino-acid position 129. The Il2ra mut cDNA was then cloned into pMIG to generate pMIG- Il2ra mut . The presence of the introduced point mutation was confirmed by sequencing. 293T cells were plated 2 days before transfection on 100 mm adherent petri dish at 10 6 cells per plates. Cells at 70% confluence were transfected with 30 µg of the plasmid pMIG, pMIG- Il2ra or pMIG- Il2ra mut using 45 µl Lipofectamine 2000 in 4.5 mL OptiMEM (ThermoFisher) overnight in antibiotic-free medium. Medium was replaced the day after transfection and 3 days later, cells were trypsinized and analyzed for CD25 extra- and intracellular expression by flow cytometry as described before. The 293T cells were a kind gift from Heather Melichar (University of Montreal, Canada) and were tested mycoplasma negative. In vitro T conv and T reg cell assays For all assays, naive CD4 + or CD8 + T conv cells were negatively selected from spleen and LNs using either anti-CD8β (H35) or anti-CD4 (GK1.5), anti-CD11b (M1/70), anti-MHC-II (M5/114), anti-TER119, anti-B220 (RA3-6B2) and anti-CD25 (PC61), all at 5 μg/mL for 30 min at 4 °C. Cells were then washed and incubated with anti-rat magnetic beads at 1 bead/target cell for 30 min at 4 °C (Dynabeads sheep anti-rat IgG, Invitrogen). For suppression assays, purified naive WT Cd45.1 +/+ CD4 + T conv cells were stained with 1–5 μM of CellTrace Violet (CTV, Invitrogen) according to the manufacturer’s protocol. 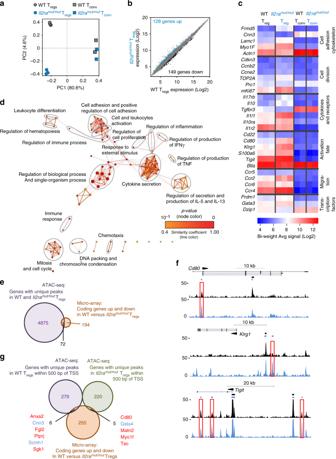Fig. 4 The expression of only a small set of genes in Tregcells is altered by low IL-2 signals:a5 × 104Tregand Tconvcells were sorted by flow cytometry from LNs of three independent replicateIl2ramut/mutor WTFoxp3Rfp/Rfpreporter mice and total RNA extracted and reverse transcribed to cDNA. Affymetrix mouse expression arrays (Pico 1.0) were then conducted. Principal component analysis (PCA) of expressed genes using the top 10% of genes with the highest variance in analyzed groups with each symbol featuring one mouse.bScatter plot of individual genes expressed inIl2ramut/mutvs WT Tregcells. Significantly upregulated and downregulated genes, defined as genes with at least 1.5 fold change,p-value ≤ 0.01, are colored blue or black, respectively, and numbers are shown.cHeat map of selected genes grouped under various categories as indicated and for which expression is significantly different betweenIl2ramut/mutand WT Tregcells.dNetwork analysis of biological-process gene-ontology (GO) term enrichment among significantly upregulated genes inIl2ramut/mutvs control WT Tregcells. Upregulated genes were analyzed for over-represented GO terms using BiNGO in Cytoscape, and the resulting network was calculated and visualized using EnrichmentMap. Groups of similar GO terms were manually circled. Line thickness and color are proportional to the similarity coefficient between connected nodes. Node color is proportional to the FDR-adjusted p-value of the enrichment. Node size is proportional to gene set size.eVenn diagram comparing differentially expressed genes inIl2ramut/mutvs WT Tregcells to genes with unique peaks called inIl2ramut/mutand WT Tregcells found in ATAC-seq in Fig.3based on gene symbols.fATAC-seq tracks for 3 sample genes with at least 1 unique peak localized in distinct regions of the gene (promotor, intronic, intergenic).gThree-way Venn diagram comparing differentially expressed genes inIl2ramut/mutversus WT Tregcells to genes containing unique peaks close to TSS (<500 bp) inIl2ramut/mutvs WT Tregcells found in ATAC-seq WT and Il2ra mut/mut Foxp3 Rfp/Rfp T reg cells were sorted by flow cytometry (Aria III). 5 × 10 4 CTV-labeled naive CD4 + T conv cells were cultured with increasing numbers of T reg cells in the presence of 10 5 irradiated, T cell-depleted WT B6 splenocytes and 1 μg/mL anti-CD3ε (clone 145-2C11, BD) in a 96 round-bottom plate for 72 h. Cell proliferation of T conv cells (live CFSE − CD4 + Foxp3 − ) was determined by flow cytometry based on CTV fluorescence intensity dilution of T conv cells. For proliferation assays, CTV-labeled purified WT and Il2ra mut/mut naive CD4 + or CD8 + T conv cells were incubated for 24 h on anti-CD3ε (10 μg/mL) pre-coated wells before co-culture for 96 h with varied concentrations (2.5-10 4 U/mL) of human recombinant IL-2 (Gemini Bio-product). Cell proliferation was determined by flow cytometry and CTV fluorescence dilution of T conv cells. For short-term activation assays for immunofluorescence, purified WT and Il2ra mut/mut naive CD4 + T cells were incubated for 48 h with anti-CD3ε (10 μg/mL) pre-coated wells to induce CD25 upregulation. At 48 h, cells were transferred in polylysine pre-coated chambers, left to adhere for 1 h at 37 °C, fixed with 1% PFA and permeabilized with 0.1% Triton X-100 prior to OVN staining in PBS 0.5% BSA, 0.05% Triton X-100 containing polyclonal goat anti-mouse CD25 (RD systems) and rabbit anti-calreticulin Abs (1/300 dilution, ThermoFisher, PA3-900). Staining was revealed by staining for 2 h with secondary anti-goat-Alexa 488 and anti-rabbit-Alexa 546 Abs (Invitrogen). Cells were then covered with Fluoromount-G (SouthernBiotech) and imaged using a Zeiss Axiovert microscope (Carl Zeiss Microimaging Inc., Thornwood, NY) with a ×63 NA 1.4 objective and a Retiga 2000 camera. 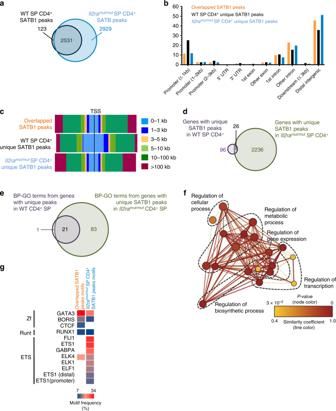Fig. 5 Ectopic DNA binding of SATB1 in SP CD4+thymocytes receiving low IL-2 signals: 2 × 106SP CD4+thymocytes were sorted in 2 independent duplicate experiments by flow cytometry from the thymus ofIl2ramut/mutand WT mice, PFA fixed, lysed, and cross-linked DNA was used for chromatin immunoprecipitation sequencing (ChIP-seq) of the pioneer factor SATB1.aVenn diagram of the number of common and unique SATB1 DNA binding peaks inIl2ramut/mutvs WT SP CD4+thymocytes.b,cDistribution of common and unique SATB1 DNA binding peaks across gene organization (b) and distance to the transcription start site (TSS,c) in the whole genome.dVenn diagram of the number of genes exhibiting unique SATB1 DNA binding peaks inIl2ramut/mutvs WT SP CD4+thymocytes.eVenn diagram of biological-process gene-ontology (BP-GO) from genes with unique SATB1 DNA binding peaks in WT vsIl2ramut/mutSP CD4+thymocytes.fNetwork analysis of BP-GO term enrichment among genes with unique SATB1 DNA binding peaks in WT SP CD4+thymocytes. Genes with unique SATB1-binding peaks were analyzed for over-represented GO terms using BiNGO in Cytoskape, and the resulting network was calculated and visualized using EnrichmentMap in Cytoscape. Groups of similar GO terms were manually circled. Line thickness and color are proportional to the similarity coefficient between connected nodes. Node color is proportional to the FDR-adjustedp-value of the enrichment. Node size is proportional to gene set size.gFrequency of known TF binding site motifs enriched in common and unique SATB1 DNA binding peaks in WT andIl2ramut/mutSP CD4+thymocytes. Motif frequency (%) is shown in heat map Green channel images using a 450–490 excitation/500–550 emission bandpass filter and red staining was imaged with a 565/30 excitation-620/60 emission bandpass filter. Images were processed using Adobe Photoshop CS 4 (Adobe Systems, Inc. San Jose, CA). In vivo T reg cell functional assays For mixed bone-marrow chimera mice , Rag1 − / − Cd45.2 +/+ mice were lethally irradiated with 1200 rads before immediate reconstitution with 5 × 10 6 T cell-depleted (as for the in vitro assays) bone marrow from Foxp3 − /y Cd45.1 +/+ and Il2ra mut/mut Cd45.1 +/ − or congenic Cd45.1 +/+ and Il2ra mut/mut Cd45.1 +/ − at a 1:1 ratio. Mice were placed under antibiotics for 2 weeks and reconstitution ratios were checked by FACS 4–6 weeks later. In some experiments, C57BL/6 Cd45.2 +/+ were used as recipient. In such case, mice received 150 μg of anti-CD8β and anti-CD4 i.v. with for two consecutive days to deplete T cells prior irradiation. For Rag1 −/− T cell transfers, LN- and spleen-purified naive CD4 + T conv cells (by negative selection as above) isolated from Cd45.1 +/+ male mice were transferred to Rag1 −/− recipients alone or mixed at a 5:1 ratio with flow-sorted sorted (Aria III) RFP + T reg cells from spleen and LNs of WT or Il2ra mut/mu t Foxp3 Rfp/Rfp reporter mice (2.5 × 10 6 cells per recipient). In some experiments (when indicated), naive CD4 + T cells were labeled with 10 nM of CTV prior adoptive transfer. Recipient mice were monitored for body weight changes and transferred lymphocyte subsets were monitored by flow cytometry 45 and 75 days later. For Foxp3 − /y mice rescue experiments, 10 6 flow-sorted T reg cells from WT or Il2ra mut/mut Foxp3 Rfp/Rfp reporter mice were injected i.p. into 1–2-day-old pups ( Foxp3 y/− males, genotyped after birth) from females Foxp3 +/ − mice bred with Cd45.1 +/+ congenic males. Male pups were assessed for the development of lymphoproliferative syndrome in blood and LNs at ~30 days of age. For the antibody neutralization treatment, mice were given 150 µg of anti-ICOSL (clone HK5.3, BioXcell) by i.v. injection on days 0, 3, 6, 9, and 12 and sacrificed on day 14. Histological analysis Tissue samples were fixed in 10% neutral buffered formalin and processed for hematoxylin and eosin staining. For each organ collected and for each genotype, two sections were cuts at 100 μm apart and all slides were scanned using a P250 High Capacity Slide Scanner (Perkin Elmer). Microarrays Overall, 50,000 RFP + T reg or naive (CD62L hi CD44 lo ) RFP neg CD25 neg CD4 + T conv cells from LNs of WT or Il2ra mut/mut Foxp3 Rfp/Rfp mice were flow-sorted based on the RFP signal and indicated markers after enrichment for CD4 + T cells (using negative selection, as described above). Pelleted cells were stored in 700 μL of TRIzol (Life Technologies) at −80 °C until RNA extraction. Total RNA was extracted using the RNAeasy Micro kit with RNase-Free DNase Set (Qiagen) according to the manufacturer protocol. The quality score and quantity of purified RNA was assessed with a Bioanalyzer RNA 6000 Pico Chip (Agilent). Total RNA was then converted to cDNA, amplified and hybridized to Affymetrix Mouse Transcriptome Array 1.0 Pico. Raw CEL files were preprocessed and normalized using Affymetrix Expression Console (version 1.4.1.46) and resulting data were analyzed with the Affymetrix Transcriptome Analysis Console (version 3.1.0.5). We calculated fold-differences between experimental groups and tested significance using one-way ANOVA (unpaired). Significantly up and downregulated genes were defined with at least a 1.5-fold expression difference and a p -value ≤ 0.01. Over-representation of biological-process (BP) gene-ontology (GO) terms was calculated using BiNGO (version 3.0.3) in Cytoscape (version v3.4.0), employing the hypergeometric test and applying a significance cutoff of FDR-adjusted p -value ≤ 0.05. The GO ontology and annotation files used were downloaded on May. 25, 2017. The output of BiNGO was imported into EnrichmentMap (version 2.1.0) in Cytoscape to cluster redundant GO terms and visualize the results. An EnrichmentMap was generated using a Jaccard similarity coefficient cutoff of 0.4, a p -value cutoff of 0.001, an FDR-adjusted cutoff of 0.005, and excluding gene sets with fewer than 5 genes. The network was visualized using a perfuse force-directed layout with default settings and 500 iterations. Groups of similar GO terms were manually circled. Finally, for analysis of gene expression in thymocyte fractions shown in Supplementary Fig. 5c , raw data from the NCBI database (GEO GSE15907) were analyzed [41] . Epigenetic profiling For ATAC-seq experiments, we performed the analysis on two (LNs) or four (thymus) biological replicates per group as previously described [35] . Briefly, nuclei were isolated from 50,000 CD4 + T cell-enriched (by negative selection) flow-sorted RFP + T reg cells from WT or Il2ra mut/mut Foxp3 Rfp/Rfp mice (LNs or thymus) using a solution of 10 mM Tris-HCl, 10 mM NaCl, 3 mM MgCl 2 , and 0.1% IGEPAL CA-630. Immediately following nuclei isolation, the transposition reaction was conducted using Tn5 transposase and TD buffer (Illumina) for 45 min at 37 °C. Transposed DNA fragments were purified using Qiagen Mini-Elute Kit and PCR amplified using NEB Next High Fidelity 2× PCR master mix (New England Labs) with dual indexes primers (Illumina Nextera). For SATB1 ChIP-seq experiments, we performed the ChIP-seq following the Mayers Lab ChIP-seq Protocol v011014 which is one of the suggested protocols by ENCODE project with slight modifications ( https://www.encodeproject.org/documents/6ecd8240-a351-479b-9de6-f09ca3702ac3/@@download/attachment/ChIP-seq_Protocol_v011014.pdf ). Single positive (SP) CD4 + thymocytes from thymus of WT and Il2ra mut/mut mice on two biological replicates were pre-enriched by negative selection using anti-CD8β (H35), anti-MHC-II (M5/114), anti-CD11b (M1/70) and anti-TER119. After staining the remaining cells with fluorescent labeled antibodies against CD4 (GK1.5) and CD8α (53-6.7), we flow-sorted 2 × 10 6 CD4 + CD8α neg SP thymocytes. Sorted cells were next cross-linked in 1% (wt/vol) formaldehyde solution for 30 min. Cross-linked DNA was lysed in Farnham lysis buffer (5 mM PIPES pH 8.0, 85 mM KCl and 0.5% NP-40), fragmented in RIPA buffer (1% NP-40, 0.5% sodium deoxycholate, and 0.1% SDS in 1×PBS) using Bioruptor (Diagenode), and incubated overnight at 4 °C with 100 µL of DynaBeads M-280 Sheep anti-Rabbit IgG magnet beads (Invitrogen) preincubated with 20 µg of anti-SATB1 antibody (Abcam, ab70004). Beads were washed five times with LiCl wash buffer (100 mM Tris pH 7.5, 500 mM LiCl, 1% NP-40 and 1% sodium deoxycholate) and one time with 10 mM Tris/0.1 M EDTA. SATB1-bound DNA was then eluted from the beads and reverse cross-linked by incubating the beads pellet in 200 µl of IP elution buffer (1% SDS and 0.1 M NaHCO 3 ) at 65 °C overnight and further purified with MinElute PCR Purification Kit (QIAGEN). The library was prepared using Accel-NGS 2 S Plus DNA library kit according to the manufacturer’s instructions. Sequencing libraries processing The size distribution and molarity of the sequencing library were determined by using an Bioanalyzer analysis (High Sensitivity DNA chip, Agilent). Sequencing was performed using a HiSeq 2500 system (Illumina). Obtained sequences were mapped to the mouse mm10 reference genome using BWA mem [57] , [58] . After eliminating duplicated reads and the reads aligned to mitochondrial DNA, we kept only concordantly mapped pairs for further analysis. Peak calling was performed on shifted reads using MACS v2.1 with narrow peaks option to identify areas of sequence tag enrichment following the original report [35] . For ATAC-seq, read1 reads were shifted using bedtools2, as previously performed in Buenestro et al. [35] , before calling peaks for each replicate. 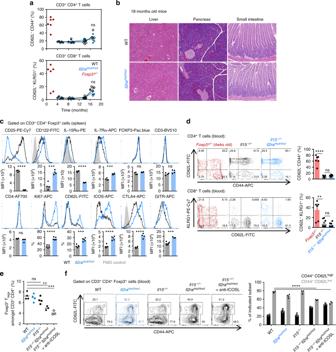Fig. 6 Il2ramut/mutmice do not develop any signs of autoimmunity:aT cells collected from blood ofIl2ramut/mutand WT mice were stained for cell-surface CD3, CD8, CD4 and CD62L, CD44, KLRG1 activation markers at indicated times over an 18 months period. Blood from controlFoxp3y/−was analyzed at ~1.5 months post birth. Each symbol represents an individual mouse.bAt month 18, liver, pancreas, and small intestine were harvested, fixed/cut, and stained with H/E.cSpleen cells from 8 to 10-weeks-oldIl2ramut/mutand WT mice were stained for cell-surface CD3, CD4, intracellular Foxp3 and indicated markers. Overlay of representative FACS histograms after gating on CD3+CD4+Foxp3+T cells are shown and bar graphs average relative expression levels (MFI,n= 4–5).dBlood fromIl2ramut/mutIl15−/−,Il15−/−(6 months old) orFoxp3y/−mice was stained as inaand representative FACS dot plots with bar graphs summarizing average across mice (n= 6–7) are shown.eProportion of peripheral blood Foxp3+Tregcells among CD3+CD4+T cells in indicated mice treated (or not) with anti-ICOSL for 2 weeks.fBlood leukocytes from indicated mice groups were stained for expression of CD3, CD4, intracellular Foxp3, CD62L, CD44. Representative dot plots and summary bar graphs of average CD44/CD62L expression levels across all groups of mice are shown (n= 3–4).p-values are indicated when relevant with *p< 0.05; **p< 0.01; ***p< 0.001; NS not significant, using two-tailed unpaired Student’st-test 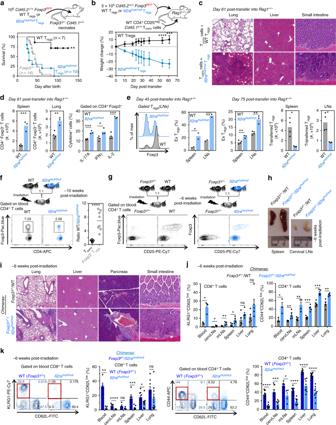Fig. 7 Tregcells receiving limited IL-2 signals cannot suppress autoreactive WT Tconvcells:aFoxp3y/−Cd45.1+/+neonate mice were transferred i.p. with 106Il2ramut/mutor WT flow-purifiedFoxp3Rfp/RfpCD3+CD4+Tregcells and survival was monitored over 120 days. Graphs average results over multiple mice in each group and 7-16 replicate experiments.b,cRag1−/−mice received 5 × 105flow-purifiedFoxp3Rfp/RfpCD3+CD4+Tregcells together with 1.5 × 106WT CD3+CD4+CD25negTconvcells i.v. Weight loss was monitored up to 61 days post transfer and immune cell infiltrates on H/E stained sections is shown at day 61 (n= 4).dNumbers of transferredFoxp3Rfp/RfpCD3+CD4+Tregcells in the spleen and lung ofRag1−/−mice (left bar graphs) and proportion of cytokine-secreting CD3+CD4+Tconvcells 4 h post PMA/ionomycin stimulation.eFoxp3 expression inFoxp3Rfp/RfpCD3+CD4+Tregcells 45 and 75 days post transfer, proportion and absolute numbers of ex-Tregcells in LNs and spleens.f,gSchematic of mixed bone-marrow chimera generation in lethally irradiated WT B6 recipient mice with discriminative congenic markers.f,gRepresentative FACS dot plots of Foxp3 and CD4 expression in blood T cells offWT/Il2ramut/mutandgFoxp3y/−/WT andFoxp3y/−/Il2ramut/mutchimeras 10 and 6 weeks post reconstitution, respectively. Graph infshows the ratio of WT vsIl2ramut/mutTconvand Tregcells for each individual chimera. Data are across several chimeras (5–9 mice/group) in 3–4 replicate experiments.h,iSpleen, LN pictures, and H/E stained sections of lung, liver, pancreas, and small intestine fromFoxp3y/−/WT andFoxp3y/−/Il2ramut/mutchimeras.jCells from indicated organs from the two groups of chimeras were stained for cell-surface expression of CD3, CD4, CD8, CD62L, KLRG1, and CD44. Bar graphs show the proportion of activated CD4+(CD44+CD62Llo) or CD8+(KLRG1+CD62Llo) T cells (n= 5–9).kProportion of activated CD3+CD4+or CD8+Tconvcells fromIl2ramut/mutor WT BM inFoxp3y/−/Il2ramut/mutchimeras. Bar graphs summarize average proportion across mice (n= 5–9). p-values are indicated when relevant with *p< 0.05; **p< 0.01; ***p< 0.001; NS not significant, using two-tailed unpaired Student’st-test. Symbols on bar graphs feature individual mice We performed Irreproducible Discovery Rate analysis for finding reproducible peaks among the biological replicates (0.05 cutoff) [59] . Analysis was performed in R (the R project) using Bioconductor packages. The genomic locations, overlapping or nearest genes and finding overlapping peaks between groups were annotated with ChIPpeakAnno [60] and ChIPseeker [61] using TxDb.Mmusculus.UCSC.mm10.knownGene annotation (Bioconductor). The motif analysis was performed on the genomic sequences of peaks using MEME-ChIP 63 and HOMER [62] . Over-representation of biological-process BP-GO terms was calculated using BiNGO as described above. For the ATAC-seq data analysis, the output of BiNGO was further filtered by selecting GO with an FDR-adjusted cutoff < 0.001 and excluding gene sets with fewer than five genes. The list of BP-GO was then imported into REViGO using a similarity coefficient of 0.7 and the SimRel columns to generate semantic similarities scores. The scored terms were visualized in semantic similarity-based scatterplots. For the SATB1 ChIP-seq data analysis, the output of BiNGO was imported into EnrichmentMap (version 2.1.0) in Cytoscape to cluster redundant GO terms and visualize the results as described above. Statistics Statistical significance was calculated using an unpaired Student t test with GraphPad Prism software and two-tailed P values are given as: (*) p < 0.1; (**) p < 0.01; (***) p < 0.001; (****) p < 0.0001 and (ns) p > 0.1. All p values of 0.05 or less were considered significant and are referred to as such in the text. Error bars are mean ± SEM in all figures.